The impact of sleep deprivation on food desire in the human brain Epidemiological evidence supports a link between sleep loss and obesity. However, the detrimental impact of sleep deprivation on central brain mechanisms governing appetitive food desire remains unknown. Here we report that sleep deprivation significantly decreases activity in appetitive evaluation regions within the human frontal cortex and insular cortex during food desirability choices, combined with a converse amplification of activity within the amygdala. Moreover, this bi-directional change in the profile of brain activity is further associated with a significant increase in the desire for weight-gain promoting high-calorie foods following sleep deprivation, the extent of which is predicted by the subjective severity of sleep loss across participants. These findings provide an explanatory brain mechanism by which insufficient sleep may lead to the development/maintenance of obesity through diminished activity in higher-order cortical evaluation regions, combined with excess subcortical limbic responsivity, resulting in the selection of foods most capable of triggering weight-gain. Mounting epidemiological data implicate sleep loss as a risk factor for obesity in both children and adults worldwide [1] . Moreover, sleep deprivation alters appetite-regulating hormones and increases caloric intake [2] , [3] . Given the continued decline in sleep duration in industrialized nations, mirrored by the steep rise in obesity in these same populations [1] , understanding the association between sleep loss and weight gain has become of paramount concern for global public health. Despite such population-level as well as peripheral body evidence, the central brain mechanisms explaining the impact of sleep deprivation on appetitive food desire that can lead to weight-gain remain unknown. Discovering such neural dysfunction may represent a critical component to understanding the link between sleep loss and obesity [2] . It would further contribute to a central nervous system explanation for the failure to appropriately regulate dietary intake and thus develop or maintain obesity under conditions of insufficient sleep. Using a food-desire task in combination with human functional MRI (fMRI), here we sought to characterize the impact of sleep loss on the brain mechanisms governing appetitive food desire. The study focused a priori on a discreet set of well-characterized cortical and subcortical regions of interest (ROIs) known to be instrumental in appetitive desire and food stimulus evaluation [4] . At the cortical level, the anterior insular cortex, lateral orbital frontal cortex and anterior cingulate cortex, all have well established roles in signalling stimulus value across contexts, including appetitive choices, and in integrating food features that govern preferences (for example, the odour and flavour of food) [5] , [6] . Moreover, disrupted functional activity within frontal cortex, including these anterior cortical regions, is widely considered to be one hallmark of sleep loss [7] . At the subcortical level, both the amygdala and the ventral striatum have been strongly implicated in governing the motivation to eat [4] . The amygdala has consistently demonstrated responsivity to food stimuli, especially when the salience of food stimuli is high [8] . Activity in the ventral striatum in response to foods accurately predicts immediate food intake [9] , binge eating [10] as well as real-world weight gain [11] . Moreover, previous work has demonstrated that activity in the amygdala and striatum in other (non-appetitive) affective tasks is elevated following sleep loss [12] , [13] . Building on this established literature, the current study sought to test two non-mutually exclusive hypotheses regarding the central brain mechanisms that may lead to weight-promoting food choices following sleep loss. One hypothesis is that failure to recruit cortical regions necessary for optimal evaluation of food stimuli (the anterior cingulate, the lateral orbitofrontal cortex and the anterior insula) leads to improper food choice selection (that is, choosing items with greater weight-gain potential). A second hypothesis is that excessive reactivity in two subcortical regions known to signal food salience and promote eating behaviour (the amygdala and the ventral striatum) may exaggerate food salience and motivated consumption for appetitive food stimuli, also leading to weight-gain potential. The findings reported here demonstrate not only reduced recruitment of all three key cortical regions necessary for food stimulus evaluation but also amplified subcortical amygdala (yet not ventral striatal) reactivity under sleep deprivation. Such changes offer a novel explanatory brain mechanism by which insufficient sleep may lead to altered food choices and thus the development or maintenance of obesity. Neural responses to food desire under sleep deprivation Compared to the sleep-rested state, sleep deprivation significantly diminished activity in all three cortical ROIs—the anterior cingulate cortex ( T =3.87; P =0.0008), lateral orbital frontal cortex ( T =2.08; P =0.0491) and anterior insular cortex ( T =2.63; P =0.0154)—as food desire progressively increased ( Fig. 1a ). This was further confirmed by t -tests of averaged parameter estimate activity extracted from 5-mm spheres placed around these literature-based ROIs (see Methods). Note that the significance threshold is P <0.05 for each region; however, if all five ROIs are considered as a family of independent tests, and correcting for multiple tests, the lateral orbital frontal cortex and anterior insula no longer survive this more stringent statistical threshold, whereas the anterior cingulate remains significant. It should be noted that the latter approach makes an assumption of independence of these regions, which may not be the case considering their collective function in appetitive processing. When considering the subcortical ROIs, the amygdala expressed a significant increase in responsivity to desirable food items following sleep deprivation ( T =3.08; P =0.0055), compared with the sleep rested state ( Fig. 1b ). In contrast, this profile of amplified subcortical reactivity was not observed in ventral striatum ( T =−0.28; P =0.7852), showing no significant difference between the sleep deprivation and rested conditions. Of note, the amygdala also survives correction for five comparisons if these regions are taken as a family of independent tests. 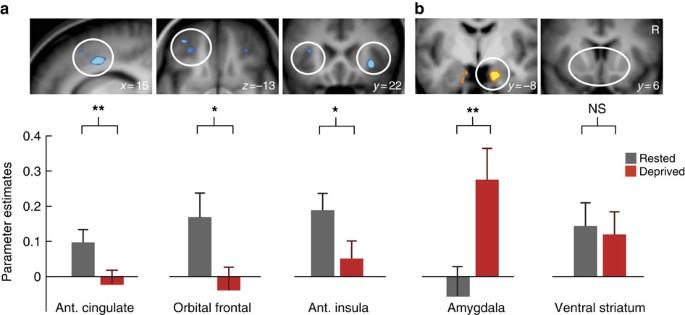Figure 1: Neural consequences of sleep deprivation on food desirability. Sleep deprivation triggered marked decreases in the anterior cingulate, left lateral orbital frontal cortex and anterior insular reactivity to food desirability (a). In addition, sleep deprivation resulted in a significant increase in amygdala reactivity to food desirability but no significant difference in ventral striatum reactivity (b). All parameter estimates are from a GLM with a parametric contrast of individual ‘want’ ratings from 23 participants. Whole-brain analysis (above) are thresholded atP<0.005 for display purposes. ROI analysis (represented by the bar graphs) are mean parameter estimates with s.e.m. extracted from 5-mm spheres centred at foci taken from previous literature (see Methods; circles indicate general areas of interest not specific foci; *P<0.05 for pairedt-tests across 23 participants and **P<0.05 with Bonferroni correction for five ROIs).Table 2reports whole-brain activation differences between sleep-rested and deprived conditions beyond oura prioriROIs (P<0.001 uncorrected using voxel-wise pairedt-tests). Error bars are represented as s.e.m. Additionally, complimenting the average activity analysis approach, described above, all ROIs of significance also demonstrated clusters of activity that survived familywise error rate correction for multiple comparisons within these small volumes ( P <0.05; Table 1 ). 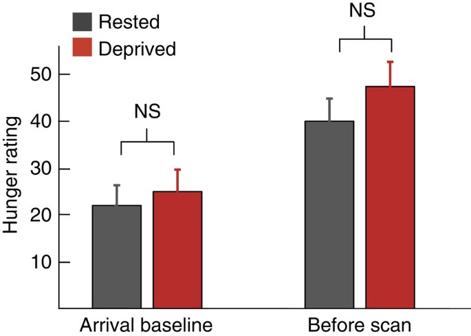Figure 2: Self-reported hunger levels. There were no significant differences between sleep-rested and sleep-deprived conditions in self-reported hunger (collected using a visual analogue scale with a 10-cm line,yaxis is in mm) either at arrival on the experimental evenings, or before the fMRI scan session in the mornings. Hunger levels were significantly greater before the scan compared with study arrival (the evening before) in both groups (P<0.05; pairedt-tests across 23 participants). Error bars are represented as s.e.m. For completeness, and as this is the first study to our knowledge to assess neural responses to food desire after sleep loss, Table 2 reports exploratory whole-brain activation differences between sleep-rested and deprived conditions ( P <0.001 uncorrected using voxelwise paired t -tests). In summary, sleep deprivation diminished activity in an established set of cortical appetitive evaluation regions as food-desire progressively increased, yet triggered a converse amplification in subcortical amygdala reactivity known to signal food salience in the context of appetitive choice [8] . Importantly, self-reported hunger levels were no different between the sleep-rested and sleep-deprived conditions ( P =0.28; see Fig. 2 ), indicating that differences in brain activity could not be explained on the basis of hunger differences alone. Figure 1: Neural consequences of sleep deprivation on food desirability. Sleep deprivation triggered marked decreases in the anterior cingulate, left lateral orbital frontal cortex and anterior insular reactivity to food desirability ( a ). In addition, sleep deprivation resulted in a significant increase in amygdala reactivity to food desirability but no significant difference in ventral striatum reactivity ( b ). All parameter estimates are from a GLM with a parametric contrast of individual ‘want’ ratings from 23 participants. Whole-brain analysis (above) are thresholded at P <0.005 for display purposes. ROI analysis (represented by the bar graphs) are mean parameter estimates with s.e.m. extracted from 5-mm spheres centred at foci taken from previous literature (see Methods; circles indicate general areas of interest not specific foci; * P <0.05 for paired t -tests across 23 participants and ** P <0.05 with Bonferroni correction for five ROIs). Table 2 reports whole-brain activation differences between sleep-rested and deprived conditions beyond our a priori ROIs ( P <0.001 uncorrected using voxel-wise paired t -tests). Error bars are represented as s.e.m. Full size image Table 1 Small volume corrections analysis. Full size table Table 2 Exploratory whole-brain analysis. Full size table Figure 2: Self-reported hunger levels. There were no significant differences between sleep-rested and sleep-deprived conditions in self-reported hunger (collected using a visual analogue scale with a 10-cm line, y axis is in mm) either at arrival on the experimental evenings, or before the fMRI scan session in the mornings. Hunger levels were significantly greater before the scan compared with study arrival (the evening before) in both groups ( P <0.05; paired t -tests across 23 participants). Error bars are represented as s.e.m. Full size image Behavioural changes in food desire under sleep deprivation Complimenting these changes in brain responsivity, we further examined whether sleep deprivation triggered an increase in desirability for food items carrying the greatest weight-gain promoting potential; that is, high-calorie food items. Relative to the sleep-rested state, sleep deprivation resulted in a significant increase in the proportion of ‘wanted’ food items of high-caloric content ( T =2.21, P =0.04). In contrast, no corresponding differences between the sleep-rested and sleep-deprived states were observed for low calorie items ( T =1.15, P =0.26; Fig. 3a ). Indeed, the total calorie content of all wanted items (summed together) in the sleep-deprived condition was significantly greater compared with the sleep-rested state ( T =2.07, P =0.05), representing an additional 600(±289 s.d.). Calorie-average increase. Additionally, the level of caloric content across food items significantly predicted the extent to which desirability ratings increased after sleep deprivation, such that the highest calorie foods accrued the largest increase in desirability ratings following sleep deprivation (Spearman’s r= 0.23, P =0.04). Further implicating an association with insufficient sleep, increasing perceived severity of sleep deprivation across individuals, indexed by self-reported subjective sleepiness [14] , was positively and significantly correlated with the percentage of wanted high-calorie foods in the sleep-deprived state ( Fig. 3b ), and this correlation remained significant when controlling for body mass index (BMI) using linear regression ( T =3.41, P =0.003). Confirming the specificity of this finding to the state of sleep deprivation, no such association between subjective sleepiness and percentage of wanted high-calorie foods was observed in the sleep-rested state ( r =0.19; P =0.39). Additionally, BMI was not correlated with the percentage of high-calorie choices in either the sleep-rested or sleep-deprived condition ( r =−0.23, P =0.30, and r =−0.05, P =0.80, respectively), consistent with previous studies examining calories from snacks rather than meals [15] . Therefore, paralleling the observed change in the neural reactivity, sleep deprivation induced a concomitant behavioural profile of increased desire for weight-gain promoting (high-calorie) food choices, with inter-individual differences in the magnitude of such a change in food choice behaviour being accounted for by the severity of perceived subjective sleepiness. 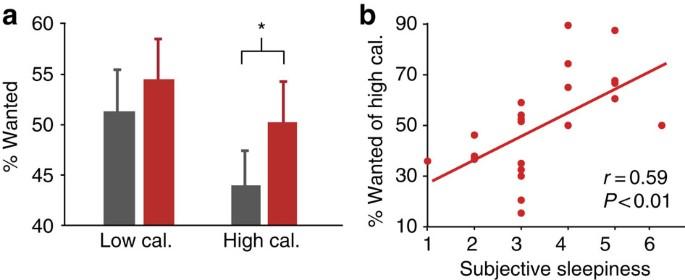Figure 3: Behavioural consequences of sleep deprivation on food desirability. Behavioural responses for the percentage of wanted high- and low-calorie items respectively (a) and the degree to which individual differences in sleepiness14(after sleep deprivation) predict wanted high-calorie choices (b). High/low calorie items are based on the median split of calories per serving; wanted items were collapsed across ‘somewhat’ and ‘strongly’ wanted ratings (*P<0.05; pairedt-test across 23 participants). Error bars are represented as s.e.m. Figure 3: Behavioural consequences of sleep deprivation on food desirability. Behavioural responses for the percentage of wanted high- and low-calorie items respectively ( a ) and the degree to which individual differences in sleepiness [14] (after sleep deprivation) predict wanted high-calorie choices ( b ). High/low calorie items are based on the median split of calories per serving; wanted items were collapsed across ‘somewhat’ and ‘strongly’ wanted ratings (* P <0.05; paired t -test across 23 participants). Error bars are represented as s.e.m. Full size image Taken together, these findings establish a disrupting impact of sleep deprivation that blunts activity in established appetitive evaluation regions [5] within the human frontal and insular cortex during food desirability choices, yet a converse subcortical amplification of reactivity within the amygdala, known to code salience in the context of food decisions [8] . Furthermore, these neural changes were associated with a significant increase in appetitive desire for weight-gain promoting (high-calorie) food items following sleep loss, the magnitude of which was proportional to the subjective severity of sleep loss across participants. In addition, these changes occurred despite participants consuming more calories during the sleep deprivation session (provided in a controlled manner in order to offset any increased energy expenditure). Moreover, participants’ self-reported hunger levels were not different in the sleep-rested and sleep deprivation session, suggesting that the condition of sleep loss, rather than metabolic need or hunger, acts as a primary factor influencing the observed changes. The characterization of these neural and behavioural changes following sleep loss may provide several explanatory insights into a central nervous system (brain) mechanism by which insufficient sleep leads to the development/maintenance of obesity. First, these data describe a profile of bi-directional change in responsivity in appetitive-relevant brain regions following sleep deprivation. All three cortical ROIs demonstrated activity reductions following sleep loss in response to increasing food desire, while one of the two subcortical target ROIs—the amygdala, associated with salience signaling of food items—expressed significant increases in response to food desirability. Interestingly, no significant differences in reactivity were observed in the classical reward region of the ventral striatum following sleep loss. It is important to note that although these brain areas do have specific and recognized functional roles in the context of appetitive food stimulus evaluation and choice, as we examined using the current task, these regions are not limited to performing such functions. For example, the anterior cingulate has been associated with conflict monitoring [16] as well as autonomic (especially cardiovascular) regulation [17] ; the orbital frontal cortex has been associated with inhibitory control [18] ; the anterior insula has been associated with interoception [19] and the amygdala has been associated with fear and arousal processing [20] . Although our interpretation of the impact of sleep loss on these regions is made within the context of appetitive food evaluation and choice, due to the nature of the task, they may nevertheless extend beyond appetitive processes, and include alterations in other functions such as those described above. Second, this collection of brain changes may not only help account for recognized shifts in dietary intake and altered food choices following insufficient sleep [3] but further reconcile potentially dissonant previous findings. Prior reports have demonstrated that sleep restriction leads to increased caloric intake following sleep loss under non-laboratory or ‘free-living’ conditions (where food selection was not fixed) [3] , fitting with impoverished mechanisms of appetitive evaluation and choice regulated by the frontal lobe as well as heightened salience signaling within the amygdala. However, such altered food choices following sleep loss can also occur without any significant change in the ratings of the hedonic qualities of food pleasantness or food desire when smelling foods directly [3] , consistent with our observations of unaltered responding in this reward-related region of ventral striatum. Furthermore, such a neural dissociation may additionally explain why some studies have failed to observe increases in caloric intake under sleep restriction when food choices are limited to small selection arrays and eating opportunities are fixed [15] , [21] , as increases in the motivated drive to eat in the absence of food choices has been primarily associated with activity in the ventral striatum (independent of the effects of sleep loss) [9] . Therefore, one plausible interpretation emerging from our data is that impoverished recruitment of cortical regions involved in appetitive choice selection following sleep loss, combined with enhanced responsivity from the amygdala, may result in improper valuation of food stimulus features, shifting behavioural choice-selection to high-calorie desirable items driven more so by salience, when food is available. The current neural observations would therefore predict that if a range of freely attainable food choices and eating opportunities are offered (as is ecologically the case in the majority of real-world situations), then the effect of sleep deprivation would lead to a significant increase in food consumption choices considered non-optimal in the context of obesity (that is, high-calorie items). Third, and congruent with these predictions, these changes in neural reactivity to food desirability under sleep deprivation were additionally accompanied by a significant shift in preferences for food items carrying the highest caloric content. While a shift in food desire ratings was observed following sleep deprivation, the controlled eating schedule of the study precluded the ability to measure actual changes in caloric intake under ad libitum (rather than controlled) food availability. Interestingly, this alteration in food desire, coinciding with changes in brain activity, is consistent with previous behavioural findings describing increases in actual caloric intake following sleep loss when ad libitum food conditions are presented [3] , [22] and increased cravings for higher caloric food categories (for example, sweet, salty and starchy foods) [23] . Given the established increase in energy needs induced by sleep deprivation [22] , [24] , [25] , the shift towards increased caloric intake and high-calorie choice preferences identified in the current experiment, supports an adaptive homoeostatic function to recover such energy expended. However, a recent study that assessed ad libitum caloric intake as well as energy expenditure in sleep-restricted humans reported increased calorie consumption beyond that which could be explained by expended energy or altered metabolic rate [22] . Moreover, this increase in calorie intake resulted in significant gains in weight. This finding leads to the hypothesis that changes in central nervous system disruption due to sleep loss, such as the alterations in appetitive brain signaling discovered in the current study, may trigger decisions that lead to increased calorie consumption in excess of energy expenditure changes, one consequence of which is weight gain. Consistent with this proposal, we additionally demonstrated that the magnitude of change (increase) in desire for high-calorie foods was positively correlated with the perceived subjective severity of sleep deprivation across participants (indexed in the measure of sleepiness). These neural and behavioral data provide indirect support linking the state of sleep deprivation, and the subjective severity of this state, to altered internal homoeostasis following extended time awake, consistent with already established alterations in other primal homeostatic functions such as metabolic balance and temperature regulation following sleep loss [26] , [27] . This may reflect a progressive deterioration in the brain and body systems that regulate and maintain optimal energy balance, one expression of which is select cortical and subcortical dysfunction leading to increases in energy consumption through heightened desire for high-calorie foods. Finally, and related to such whole-organism considerations, elegant work has characterized peripheral body changes in appetite and metabolism-regulating hormones following sleep loss that can lead to weight-gain [2] , [26] , [28] . Our findings help establish a pattern of central nervous system dysfunction that stands alongside these peripheral body changes following sleep deprivation that, together, may converge on a common impact of sleep loss on weight-gain potential. An important next step will be to examine whether these peripheral and central nervous system pathways of sleep loss-dependent dysfunction actively interact, thus providing the first whole-organism mechanistic account underlying a relationship between sleep loss and obesity. Beyond the implications stated above, it is important to note that the current findings should be considered in the context of several limitations. First, this study used a carefully controlled feeding schedule that was standardized across participants, which did not allow us to assess actual changes in calories consumed due to sleep deprivation (although, refer to the studies by Brondel et al. [3] and Markwald et al. [22] ) or to assess the relationship between neural responses and behavioural shifts in actual calories consumed. Furthermore, due to this limitation, it will be important for future studies to assess whether access to ad libitum high-calorie food would normalize the observed brain responses under sleep deprivation potentially due to reduced motivational demands for high-calorie items after consumption. Second, all scan sessions for this study took place during the morning. As both appetite and sleep patterns are significantly influenced by circadian phase [29] , future studies will be needed to examine the interactions of measurements at different circadian phases. Indeed, recent behavioural studies indicate that the largest impact of sleep loss on altered food choices occurs during the evening [22] , [30] , leading to the prediction that changes observed in the current study would be further exaggerated when repeated later in the day. Finally, it should be noted that assessments were measured in a group of healthy young and lean participants (20.5±1.8 s.d. years of age; 23.0±1.8 s.d. BMI). An important future challenge will be to examine whether similar alterations caused by sleep deprivation are expressed across a broader age and body mass range, which is pertinent considering that hormones, metabolism as well as neural responses change over the lifespan [31] , and across a spectrum of lean-to-obese ranges [32] . In summary, these findings provide a novel brain mechanism by which sleep loss may lead to the development and/or maintenance of obesity through the selection of foods carrying obesogenic (weight-gain) potential, helping to explain the significant association between reduced sleep time and obesity reported in population-level studies [1] . They further emphasize the role of sufficient sleep as a mechanistic factor promoting weight control, one pathway of which appears to be the regulation of central brain mechanisms governing appropriate food choices. Experiment overview Twenty-three healthy participants (13 female; age: 20.5±1.8 s.d. ; BMI: 23.0±1.8 s.d.) underwent a repeated-measures, counterbalanced cross-over design involving a night of normal rested sleep (average 8.2 h asleep) and a night of monitored total sleep deprivation (average 24.6 h awake), separated by at least 7 days. Participants ate a controlled snack (see eating schedule procedures) at 0230, hours in the sleep deprivation condition that contained a calorie amount sufficient to alleviate increased energy demands estimated to be expended due to staying awake. Together with a standardized breakfast in both conditions in the morning, this eating schedule resulted in hunger ratings (measured on 100-mm visual analogue scale [23] ) that did not differ statistically ( P =0.28) between sleep-deprived (47.7±25.53 mm s.d.) and rested conditions (39.7±24.0 mm s.d.) preceding the MRI scan sessions ( Fig. 2 ). During each fMRI session (scan time 0929, hours±49 min s.d. ), participants rated 80 different food items that varied in calorie content on a 1–4 rating scale, according to how much they wanted that item ‘right now’ ( Fig. 4 ). fMRI BOLD signal was correlated with these 1–4 ratings on a trial-to-trial basis, resulting in neural activation maps expressly sensitive to increasing food-choice desire. After the scan, participants actually received one food item based on their ratings, enhancing ecological incentive context and potentially reducing demand characteristics. This paradigm therefore allowed simultaneously monitoring of behavioural food choice desire and the identification of brain areas underlying these appetitive decisions, modelled and hence sensitive to increasing food desire. 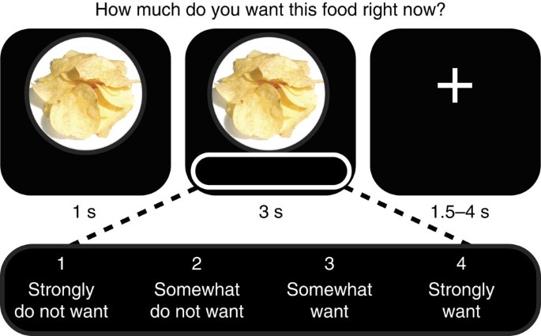Figure 4: Food-desire task trial structure. Participants saw and rated 80 food items on a scale from 1–4 according to how much they wanted the food item at that moment under sleep-rested and sleep-deprived conditions. Figure 4: Food-desire task trial structure. Participants saw and rated 80 food items on a scale from 1–4 according to how much they wanted the food item at that moment under sleep-rested and sleep-deprived conditions. Full size image Participants The Institutional Review Board of the University of California, Berkeley, approved the experimental protocol, and we obtained written informed consent from participants. Participants were free from general medical, neurological, psychiatric or sleep disorder diagnoses and did not report any history of drug abuse or head trauma. Further, participants were free from MRI contraindications, and no individual had dietary restrictions or food allergies to any of the food stimuli. Participants abstained from drugs, alcohol and caffeine for 3 days before each session. Twenty-three participants were included in the analysis (13 female; mean age: 20.5±1.8 s.d. ; mean BMI: 23.0±1.8 s.d. ; 1 participant was left-handed). Three participants (from 26 original) were excluded due to (1) failure to keep the sleep schedule (>2 h deviation), (2) initiating a gluten-free diet and (3) inability to stay awake during the deprivation scan session as evident from online eye-tracking and omitting responses on 30% of trials. The remaining participants omitted 3.9±4.3 s.d. trials under sleep deprivation and 0.2±0.4 s.d trials when rested, all separately modelled as omitted trials in the fMRI analyses. Sleep condition procedures Participants completed two experimental sessions: (1) a night of normal sleep in the lab monitored by polysomnography (PSG) and (2) a night of total sleep deprivation monitored by lab personnel (from 2100, hours) and by wrist actigraphy. Sessions were separated by a minimum of 7 days (average 10 days) and counter-balanced in order across participants. Participants completed fMRI scanning sessions the morning after each experimental night, starting at 0908, hours±45 min (range: 0805–1039, hours) on the sleep deprivation day and 0950, hours±45 min (range: 0817–1100, hours) on the sleep-rested day. To ensure that participants were well rested before each session, they kept a regular sleep schedule (7–9 h time in bed between 2200 and 1000, hours) for 3 days prior to each session, verified by daily sleep diaries and wrist actigraphy. Subjects attained 8.08±1.0 hours (s.d.) in bed across the three nights proceeding the sleep deprivation and 8.07±1.0 hours (s.d.) preceding the sleep-rested condition. Additionally, on these 3 days, participants used 5-point scales (1 indicating low/poor and 5 indicating high) to rate their subjective overall sleep quality (3.91±0.9 s.d. before sleep deprivation; 3.80±0.9 s.d. before sleep-rested), how alert they felt (3.69±0.7 s.d. before sleep deprivation; 3.63±0.8 s.d. before sleep-rested) and how well rested they felt (3.78±0.9 s.d. before sleep deprivation; 3.75±0.8 s.d. before sleep rested). Finally, participants rated their subjective sleepiness [14] as 2.09±0.9 s.d. at their arrival in the rested session ( ∼ 2000, hours) and as 2.35±1.1 s.d. at their arrival in the sleep deprivation session ( ∼ 2100, hours). Taken together, these measures suggest that participants were well rested when entering both experimental sessions. Sleep monitoring and recording procedures On the sleep deprivation experimental night, subjects were monitored using wrist actigraphy throughout the day and then additionally monitored in the lab by lab personnel, starting at 2100, hours. On the experimental night in the sleep-rested session, PSG sleep monitoring was recorded in the laboratory using 19-channel electroencephalography (EEG) (locations according to international 10–20 system), together with electro-oculography at right and left outer canthi and electromyography via three chin electrodes [33] . Sleep-staging was performed in accordance with standardized techniques [34] from the C3–A2 electrode derivation. During this PSG rested session, subjects obtained an average of 8.2±0.84 hours (s.d.) time asleep (min and s.d. ): 48.68±20.1 NREM Stage 1; 251.1±39.6 NREM Stage 2; 83.58±28.9 NREM slow wave sleep (Stages 3 and 4); 110.1±28.7 REM sleep. Eating schedule procedures Participants ate according to their normal diet throughout enrolment. During the sleep deprivation night, participants were provided with a controlled snack from 0230–0300, hours. This consisted of calorie content sufficient to offset increased energy expenditure associated with one night of sleep loss over a 24-h period (reported as 134±2.1 s.d. Cal) [24] . The snack contained the following four items: Fig Newtons (200 Cal), Gold Fish crackers (130 Cal), Ritz peanut butter crackers (150 Cal) and an apple (95 Cal), resulting in a total of 575 Cal available. On average, participants ate an estimated 485.2 Cal, with the least amount of calories consumed being ∼ 160 Cal; this was the only participant who consumed <300 Cal. Note that these estimates are based on calories per serving reported on the packaging and the proportion of the serving eaten by the participants (reported as none, half or the entire item). In addition, and in both sessions, all participants were given, and consumed, a small breakfast (one piece of toast with strawberry jam) ∼ 45 min before their scan session. Participants were monitored throughout both sessions to ensure that they did not eat anything in addition to this provided food (although water was not restricted). Self-reported hunger levels (assessed on a 100-mm visual analogue scale [23] ) immediately preceding the scan session were no different between the rested and deprived conditions ( P =0.28; also reported in Results). Both groups showed an increase in hunger levels compared with their study arrival baseline ( Fig. 2 ), which is important when considering previous studies have shown that brain reactivity to food stimuli can be enhanced by subjective hunger [35] . Food-desire task In the food-desire task, participants saw 80 food items and rated them on a 1–4 scale according to how much they wanted that food right now (details provided in Fig. 4 ). In order to control for lateralized motor effects, approximately half of the participants used their left hand to rate wanted items (1—strongly want; 2—somewhat want; 3—somewhat do not want; 4—strongly do not want) and the other half used their right hand (scale reversed). For all analyses, ratings were re-coded so that higher ratings indicated higher wanting. Participants were not informed of the hypotheses of the study nor were they told that they would be seeing foods that experimentally varied in terms of calorie content or food types that could otherwise establish preconceived biases. In the task instructions, participants were informed that two food items would be revealed at the end of the scan, and a serving of whichever item they had rated as wanting more would be given to them to eat (which was carried out). They were further instructed that this meant it was in their best interest to rate each food item according to how much they actually wanted that item at the time of the session. This procedure was used to encourage participants to rate the food items according to their actual preferences (rather than according to experimental expectations or demand characteristics), and to ensure incentive compatibility in the task as in previous studies [36] . Stimuli The task used 80 pictures of food with no packaging collected from internet searches and cropped to standardized circles. The items were evenly distributed across five categories (salty, sweet, starchy, fruit or dairy) and varied in calorie content (range: 7.2–523.4; mean: 139.8±94.8 s.d. Cal per serving based on USDA database listings ( ndb.nal.usda.gov )). The same 80 food items, but a different picture of each item, were used in each experimental session. fMRI scanning acquisition Blood oxygenation level-dependent contrast functional images were acquired with echo-planar T2*-weighted (EPI) imaging using a Siemens 3 Tesla MRI scanner with a 12-channel head coil. Each image volume consisted of 32 ascending 3.5 mm slices (96 × 96 matrix; TR=2000, ms; TE=28 ms; voxel size 2.5 × 2.5 × 3.5 mm, FOV 224 mm, flip angle=90°). One high-resolution, T1-weighted structural scan was acquired at the end of the sleep-rested session (256 × 256 matrix; TR=1900; TE=2.52; flip angle=9°; FOV 256 mm; 1 × 1 × 1 mm voxels). Concurrent eye tracking was utilized in order to further verify wakefulness. Each session was split into two 40-trial scanner acquisition runs. fMRI scanning preprocessing Preprocessing and data analysis were performed using Statistical Parametric Mapping software implemented in Matlab (SPM8; Wellcome Department of Cognitive Neurology, London, UK). First, scan-to-scan variance was assessed for quality assurance using time-series difference analysis ( http://imaging.mrc-cbu.cam.ac.uk/imaging/DataDiagnostics ) and individual scans with supra-threshold shifts (indicating high subject movement) were removed and replaced with the average of surrounding scans; these time-points were modelled out with dummy regressors (this affected six subjects). Images were then slice time-corrected, the time series was linearly detrended, then motion-corrected, smoothed using a 6-mm full-width-at-half-maximum Gaussian kernel and finally time-series were high pass-filtered (width of 128 s). General linear model A separate general linear model was constructed for each subject that included (1) all trial onsets convolved with a canonical hemodynamic response function with a 3-s duration, (2) a parametric regressor of the individual want ratings (1–4) for each food item convolved with a canonical hemodynamic response function with a 3-s duration (this was the regressor of interest) and (3) the six movement-related covariates (three rigid-body translations and three rotations determined from the realignment preprocessing step). Separate regressors were used within the same model for each of the two scanner acquisition runs. ROI analysis Guided by suggested ROI-reporting policies [37] , [38] , ROIs were taken as the average parameter estimates from 5-mm spheres centred around coordinates from previous literature examining food evaluation for the three cortical ROIs as well as the amygdala, and reward responsivity for the ventral striatum. MNI Coordinates [ x , y and z ] were: amygdala (18, −12 and −22) [8] ; ventral striatum (−12, 12 and −10) [39] ; anterior cingulated cortex (15, 6 and 38) [40] ; lateral orbital frontal cortex (−36, 42 and −10) [41] ; and bilateral anterior insula (−31, 22, 11 and 36, 17, and 0) [42] . Behavioural comparisons Behavioural comparisons between rested and deprived conditions were carried out using paired t -tests. Correlation analysis was used for results in Fig. 3b . Spearman’s correlation analysis was used to investigate the relationship between calories across food items with the mean change in desire ratings across items. How to cite this article: Greer, S.M. et al. The impact of sleep deprivation on food desire in the human brain. Nat. Commun. 4:2259 doi: 10.1038/ncomms3259 (2013).